Fast ultrahigh-density writing of low-conductivity patterns on semiconducting polymers The exceptional interest in improving the limitations of data storage, molecular electronics and optoelectronics has promoted the development of an ever increasing number of techniques used to pattern polymers at micro and nanoscale. Most of them rely on atomic force microscopy to thermally or electrostatically induce mass transport, thereby creating topographic features. Here we show that the mechanical interaction between the tip of the atomic force microscope and the surface of π -conjugated polymeric films produces a local increase of molecular disorder, inducing a localized lowering of the semiconductor conductivity, not associated to detectable modifications in the surface topography. This phenomenon allows for the swift production of low-conductivity patterns on the film surface at a speed exceeding 20 μm s −1 ; paths have a resolution in the order of the tip size (20 nm) and are detected by a conducting-atomic force microscopy tip in the conductivity maps. Multicomponent organic thin films exploiting conjugated polymers are being investigated as candidates for optoelectronic devices [1] , [2] , [3] , [4] , [5] , [6] . Among them, poly(3-hexylthiophene (P3HT)/(6,6)-Phenyl-C71-butyric acid methyl ester (PCBM) blend films are suitable in photovoltaic applications, with photoconversion efficiencies of up to 5% over small areas [7] . Owing to the interpenetrating microphase-separated internal structures, these devices are usually described as bulk heterojunction solar cells. According to the frontier energy levels of these materials, P3HT is the electron donor and PCBM is the electron acceptor; in solar cells, the P3HT absorbs in the visible part of the spectrum, generating excitons that are dissociated at the donor/acceptor interfaces [5] . In the interpenetrating network, holes move along the P3HT phase and electrons along the PCBM phase, up to collection at the electrodes. Thus, the performance of organic photovoltaic blends is affected by the film morphology that influences charge generation and transport properties [8] . Moreover, the intrinsic mobility is heavily related to the molecular order of each component of the blend, and therefore the nanoscale structure of organic solar cells has been investigated using several different microscopy techniques [9] . Among the techniques used, C-AFM (conductive-atomic force microscopy) is a scanning probe technique that allows to measure simultaneously the surface topography and the electrical properties of a sample with nanometric resolution. In details, C-AFM provides a way to perform estimations of important parameters, such as local hole and electron mobility [10] , and highlighting the relative size of donors and acceptor domains. In C-AFM, a sharp metal-coated tip is scanned across the sample, and the short-range tip–sample interaction is used as a feedback control to monitor the tip–sample distance. In its simplest application, the tip is in contact with the sample and the feedback ensures that the tip exerts a constant force. In this mode, the tip also acts as a nanoelectrode, thereby recording the current when the sample is biased with respect to the tip. Most importantly, all standard measurements supported by AFM can be carried out simultaneously (friction force—longitudinal and transverse, force-distance spectroscopy, topography and so on). In view of using polymers in organic electronics, an ever increasing number of techniques used to pattern polymers at micro and nanoscale is being promoted [11] , some directly involving AFM devices. Although most of these techniques are based on selective removal, oxidation or deposition of polymers, electrostatic nanolithography based on AFM [12] , [13] exploits the electrostatically induced mass transport of polymer, thereby creating micrometric topographic features within time scales spanning from milliseconds to seconds. In this work, we show that the mechanical friction of the AFM tip can be used to modify the local molecular order on the film surface of several conjugated polymeric semiconductors and of their blends, and in particular in the prototype photovoltaic organic blend P3HT:[70]PCBM, inducing an immediate reduction of the local carrier mobility. The increase in local disorder is demonstrated by lateral force (LF) [14] , [15] images and modelled in the framework of the Gaussian disorder model [16] . The effect results in a non-topographic high-resolution patterning of the polymer. Non-topographic patterning It is known that AFM, in contact mode, may easily abrade soft surfaces. However, in several classes of polymers, AFM-induced plastic deformations, which appear as surface nanoripples, were related to second-order phase transitions (glass-to-rubber) [17] . In the specific case of polymeric P3HT:[70]PCBM blends, we have found that the phase transition induced by the sliding AFM tip results in locally disordered (amorphous) regions where the conductivity appears heavily reduced. Interestingly, this happens even when the topographical modification only results in a marginal change in roughness (in the order of 0.1 nm r.m.s. or less) or there is no detected modification. In particular, we have spun 100-nm-thick P3HT:[70]PCBM films onto indium tin oxide (ITO), and annealed these samples at different temperatures (ranging from 100 to 200 °C) below the melting temperature of pure P3HT, which is ca. 225 °C. C-AFM measurements were performed in the configuration shown in Fig. 1a . 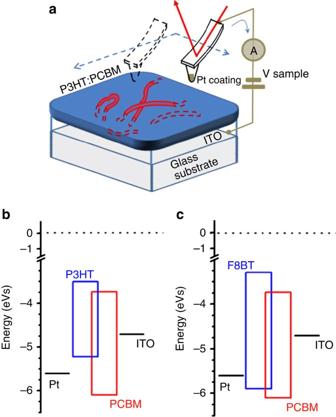Figure 1: C-AFM measurement. (a) shows our measurement set-up; (b) highlights highest occupied molecular orbital (HOMO) and lowest unoccupied molecular orbital (LUMO) energy levels of P3HT and PCBM compared with the work functions of Pt and ITO (referenced with respect to a vacuum)10, whereas (c) highlights HOMO and LUMO levels for F8BT:PCBM. Note that in our set-up, the AFM tip was grounded and the ITO was negatively biased in reverse bias mode or positively biased in the forward bias mode. Accordingly, the measurement set-up allowed to record basically hole-based currents in P3HT:PCBM. In fact, in the low reverse bias regime electron injection from ITO to the LUMO levels of P3HT and PCBM is negligible because of the very high energy barrier, unless electron tunnelling occurs. Moreover, hole injection from Pt to the HOMO of P3HT is favoured, resulting in the hole current of the device. Figure 1b also shows the typical energy levels of the samples with respect to the microscopy set-up. Figure 1: C-AFM measurement. ( a ) shows our measurement set-up; ( b ) highlights highest occupied molecular orbital (HOMO) and lowest unoccupied molecular orbital (LUMO) energy levels of P3HT and PCBM compared with the work functions of Pt and ITO (referenced with respect to a vacuum) [10] , whereas ( c ) highlights HOMO and LUMO levels for F8BT:PCBM. Note that in our set-up, the AFM tip was grounded and the ITO was negatively biased in reverse bias mode or positively biased in the forward bias mode. Accordingly, the measurement set-up allowed to record basically hole-based currents in P3HT:PCBM. In fact, in the low reverse bias regime electron injection from ITO to the LUMO levels of P3HT and PCBM is negligible because of the very high energy barrier, unless electron tunnelling occurs. Moreover, hole injection from Pt to the HOMO of P3HT is favoured, resulting in the hole current of the device. Full size image A non-topographic ‘writing’ effect was achieved by performing an AFM scan without applying any bias ( Fig. 2 ), hence without any electrostatic field or thermal excitation. Indeed, subsequent scans highlighted the previously scanned area as a region with lower conductivity. The size of the patterns (20 nm wide) is in the order of the size of the AFM tip, and patterns appear immediately. Owing to this origin, patterns are stable and, in the limit of the polymer deterioration, permanent. 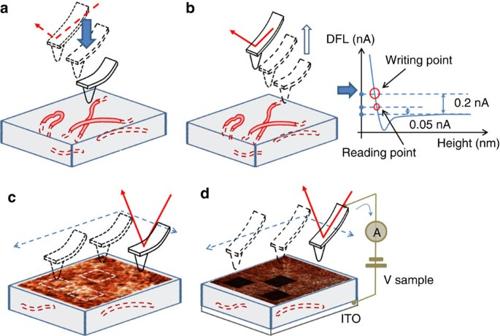Figure 2: The process of writing and reading. (a) The tip is approached to the surface in contact mode. (b) Definition of the writing and reading points through the spectroscopic curve deflection (DFL) versus height: the reading point is as close as possible to the limit where the tip stops interacting with the surface. (c) Scanning the surface in contact mode (writing). (d) Scanning the surface in spreading resistance mode (reading): reduction of the conductivity of written patterns is clearly visible. Figure 2: The process of writing and reading. ( a ) The tip is approached to the surface in contact mode. ( b ) Definition of the writing and reading points through the spectroscopic curve deflection (DFL) versus height: the reading point is as close as possible to the limit where the tip stops interacting with the surface. ( c ) Scanning the surface in contact mode (writing). ( d ) Scanning the surface in spreading resistance mode (reading): reduction of the conductivity of written patterns is clearly visible. Full size image To test patterning stability, we have created a feature, which appeared unmodified after 5 days. We have observed the phenomenon in thin films of several conjugated polymers and their blends, such as P3HT, P3HT:[70]PCBM, poly(9,9-dioctyl-fluorene-co-benzothiadiazole; (F8BT)):[70]PCBM, blends involving P3HT with different molecular weight (Mw) and blends of P3HT:[70]PCBM annealed at different temperatures. Depending on the mobility, on the band structure in our measurement set-up and on the thermal history of samples, the detection of the mobility reduction was more or less easy. The phenomenon was particularly evident and easily detectable for P3HT:[70]PCBM; as also discussed in the Supplementary Note 1 and 2 , this is because of a number of different factors; among them, there is likely the low glass-transition temperature of P3HT [18] and the relatively high order of P3HT crystallites. The molecular disorder in fact is directly related to the variance of the energy profiles of the density of states (DOS); in blends, there is also an additional effect induced by the amount and the orientation of the dipole moments in the system [19] as interface dipoles are formed at the P3HT/PCBM heterojunctions. A relevant additional factor is that the measured current may heavily depend on the metal used for the tip coating and the conductive substrate. In fact, the resulting band structure of the system tip/blend/substrate will occasionally create diode-like junctions. This is, for example, the case of F8BT:[70]PCBM blend deposited on ITO-coated glass and measured by a platinum-coated tip ( Fig. 1c ) where a potential barrier appears between tip and sample making difficult to detect the effect of writing ( Supplementary Fig. S1 ). 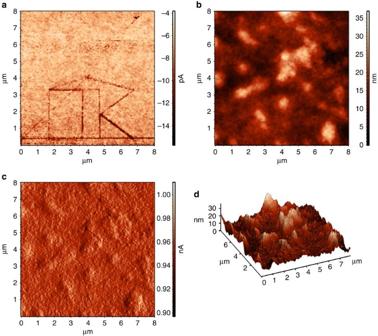Figure 3: Non-topographic writing. (a) Current map showing the pattern ‘ok’ that we have created by simply moving the AFM tip in contact with P3HT:[70]PCBM annealed at 200 °C (note: the current map has a negative offset). (b) Simultaneous topography (corrected for flattening) where there is no trace of the writing. (c) Deflection (error) image where possible scratches would be easier to detect. (d) Topography in three-dimensional images displaying no correspondent topographic effect. Figure 3a , reporting a zero bias current map for a region of the P3HT:[70]PCBM where we had previously driven the C-AFM tip along a vector path to write the word ‘OK’, shows clearly the patterning effect. As anticipated, the topography reported in Fig. 3b (in three dimensions) and the error image ( Fig. 3c ) do not show any topographic trace of such a writing, in spite of a relatively regular and flat surface. Figure 3: Non-topographic writing. ( a ) Current map showing the pattern ‘ok’ that we have created by simply moving the AFM tip in contact with P3HT:[70]PCBM annealed at 200 °C (note: the current map has a negative offset). ( b ) Simultaneous topography (corrected for flattening) where there is no trace of the writing. ( c ) Deflection (error) image where possible scratches would be easier to detect. ( d ) Topography in three-dimensional images displaying no correspondent topographic effect. Full size image The reading process involved in Fig. 3a–d is simply a further scan with a lighter set point, according to what summarized in Fig. 2 . The AFM tip is driven near the threshold where the tip is no longer in contact with the sample to ensure that no overwriting happens. In annealed P3HT:[70]PCBM, some small current was recorded in non-written areas even with nominal zero voltage bias so that maps of currents showed clearly the writing without the need of bias ( Fig. 3a is at nominal zero bias). Measurements by an oscilloscope confirm that nominal zero bias corresponds to a couple of mV of offset in the instrument (NT-MDT P47 microscope) with an amount of electrical noise, sufficient to read clearly the stored information. Owing to the work function of platinum ( Fig. 1b ) when the Pt tip serves as an electrode, the J–V curves of the P3HT:[70]PCBM films on ITO are equivalent to those of a hole-only device. In such a configuration, low-voltage current maps in P3HT:PCBM are basically hole current images and the best reading is obtained with very low bias; indeed, when increasing the bias, the current map shows the sample inhomogeneity, in particular highlighting, as expected [10] , either P3HT (bright regions)- or PCBM (dark regions)-rich domains and partly hiding the written features ( Supplementary Fig. S2 ). By using a soft tip, the CSC17/Pt/AlBS from Mikromasch, having typical force constant 0.15 N m −1 (range 0.05–0.3 N m −1 ), we were able to estimate from the deflection/distance spectroscopy ( Supplementary Fig. S3 , as example) the minimum interaction allowing a visible writing in the order of 1 nN or less. This value depends also on the annealing temperature of the samples, as the mechanical properties of the surface are also related to the thermal history of sample. Multiple reading can be achieved by using soft tips and very light set points in the feedback chain. Once writing happens, the change in conductivity is slightly modulated within 2–3 nN of force (that is, a higher contrast in the current maps may be obtained by slightly increasing the writing set point, hence the load). A further increasing of the tip pressure does not improve the writing contrast, as the low-bias conductivity is dramatically reduced, but can only lead to damages on the sample surface and to lithographic changes ( Supplementary Fig. S4 ). A moderate bias does not affect the writing effect. This is shown in Fig. 4a , reporting the current map in a region where three squares were written at different biases (−0.5, 0 or +0.5 V). On the other hand, a large bias, in the order of several volts, may induce a sharp increase of current up to several nA, triggering the melting and (relatively slow) shaping effects. We believe that this is the effect described by Zaniewski et al. [13] , where the biasing electric field induces a polymer ordering and a corresponding increase of conductivity. In our case, the writing corresponds to a lowering of the polymer conductivity, as shown in Fig. 4b , where average I–V curves (10 measurements)—along with s.d.—are evaluated inside and outside a written area in an argon-saturated atmosphere. As matter of fact, scans were performed either in air or in argon-saturated atmosphere. Although quantitative measurements of current–voltage characteristics are more reliable in controlled atmosphere, the writing process was unaffected, ruling out a possible impact of the room moisture —inducing a water meniscus between tip and sample—or tip-induced oxidation. 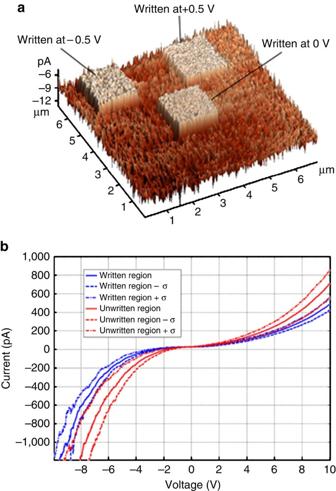Figure 4: Effect of biasing of the AFM tip. (a) Display of a current map (image reverted for clarity) showing three lower conductivity squares, created by performing three writing with different biases (P3HT:[70]PCBM annealed at 100 °C); apparently, different biases did not affect the writing process. (b) Average (and s.d.) I–V curves for written and unwritten regions (sample P3HT:[70]PCBM annealed at 100 °C). The written region results in reduction of conductivity. Figure 4: Effect of biasing of the AFM tip. ( a ) Display of a current map (image reverted for clarity) showing three lower conductivity squares, created by performing three writing with different biases (P3HT:[70]PCBM annealed at 100 °C); apparently, different biases did not affect the writing process. ( b ) Average (and s.d.) I–V curves for written and unwritten regions (sample P3HT:[70]PCBM annealed at 100 °C). The written region results in reduction of conductivity. Full size image For the sake of completeness, samples at different annealing temperatures were characterized in terms of I–V curves; the behaviour of the curves confirms the expected beneficial effect of the annealing with respect to carrier mobility ( Supplementary Fig. S5 , measurement in air), inducing the segregation of the P3HT and [70]PCBM components in well-ordered domains. Modelling The writing phenomenon is well accounted for in the framework of the extended Gaussian disorder model (EGDM) proposed in [16] . Such a model is based on the numerical solution of the master equation for hopping transport, assuming a disordered energy landscape with a Gaussian DOS and provides estimation of the mobility as a function of the electric field, of the carrier density and of the temperature (see Methods for details; Supplementary Fig. S6 for temperature behaviour). We have also obtained average—field-independent—mobility values [20] ranging from 0.0001 (as spun sample) to 0.012 cm 2 V −1 s −1 (annealed) ( Supplementary Fig. S7 , Supplementary Note 1 ). In such calculations, a slightly increased effective contact area, accounting for the surface spreading of the current, was used for the AFM tip, overcoming a potential overestimation of the actual value [21] of mobility. Consequently, the obtained values agree quite well to the values reported in the literature [10] ( Supplementary Fig. S7 ). Most importantly, we always observe a significant reduction in mobility in written regions (for example, from the original value of 0.012—unwritten—to 0.005 cm 2 V −1 s −1 ), which is well described by a slight broadening of the width of the Gaussian DOS, ranging in a fraction of eV, consequent to the induced molecular disorder. To experimentally ascertain that the reduction in conductivity can be related to the increase in the molecular disorder of the polymeric surface, we have used the LF (or friction) imaging. Basically, during the scan, the twisting of the AFM cantilever is simultaneously mapped. LF and its variant, the transverse shear microscopy, have been demonstrated to be powerful tools to investigate crystallographic features of surfaces [14] , [15] . In particular, the amorphous versions of any polymer feature a larger number of molecular-scale degrees of freedom than their crystalline counterparts. Thus, the translational kinetic energy of a sliding AFM tip is transferred to a large number of molecular motions, and modes for this to occur are larger in amorphous domains because of the greater molecular freedom. The consequence is that a region with lower molecular order will appear as a brighter region in LF scans. This is actually what happens in our case. 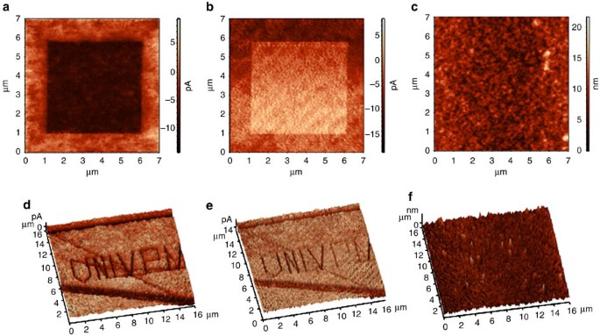Figure 5: Comparison between current maps, LF and topographic images. A square, 5 μm of side, was written; reading is performed in an area 7 × 7 μm2in P3HT:[70]PCBM (1:1) annealed at 100 °C for 15 min. (a) Current map (0.5 V). (b) LF image: the written square appears as a region with increased molecular disorder. (c) Topography: no topographic change is visible. The above images were obtained simultaneously. In addition, the acronym ‘UNIVPM’ is written and represented in three dimensions: (d) current map, (e) LF (inverted for clarity) and (f) topography. Figure 5 shows a square that was written on P3HT:[70]PCBM, appearing not only in current images (Fig. 5a) but also as a bright region in LF image (Fig. 5b) and being invisible in topography (Fig. 5c). The effect is also represented in three-dimensional mode by writing the acronym ‘UNIVPM’ in current (Fig. 5d), LF (Fig. 5e) and topography (Fig. 5f). We were not able to see the same effect in some other materials, such as poly(4,8-bis-substituted-benzo(1,2-b:4,5-b′)dithiophene-2,6-diyl-alt-4-substituted-thieno(3,4-b)thiophene-2,6-diyl) (PDBTTT) and its blend with the electron-accepting molecule of N , N ′-bis(1-ethylpropyl)-perylene-3,4,9,10-tetracarboxylic diimide (PDI), as demonstrated in Supplementary Figs S8 and S9 and discussed in the Supplementary Note 2 . PBDTTT:PDI is alternative to P3HT:PCBM in current research for organic photovoltaic cells. Figure 5: Comparison between current maps, LF and topographic images. A square, 5 μm of side, was written; reading is performed in an area 7 × 7 μm 2 in P3HT:[70]PCBM (1:1) annealed at 100 °C for 15 min. ( a ) Current map (0.5 V). ( b ) LF image: the written square appears as a region with increased molecular disorder. ( c ) Topography: no topographic change is visible. The above images were obtained simultaneously. In addition, the acronym ‘UNIVPM’ is written and represented in three dimensions: ( d ) current map, ( e ) LF (inverted for clarity) and ( f ) topography. Full size image Images were also obtained in semicontact mode (see Supplementary Figs S10 and S11 , Supplementary Note 2 ) to further investigate surface modifications, and highlighting the fibril-like P3HT crystals in the surface, agreeing with previously reported in TEM microscopy study [22] , [23] . Note that in this scanning mode, the AFM tip does not ‘write’, demonstrating that friction triggers the formation of the disordered molecular layer. In this mode, also phase images are available ( Supplementary Fig. S12 ); although phase images are always difficult to interpret, being critically dependent by several concurrent parameters, they also show to some extent the existence of the amorphous layer. In this work, we demonstrate a novel ‘nanowriting’ effect for several semiconductor polymers and blends, particularly efficient in P3HT:[70]PCBM films where a sliding AFM conductive tip induces local changes in the polymer conductivity not associated to visible topographic changes. The width of the written paths is in the order of the curvature radius of the AFM tip; patterns appear almost immediately and their creation does not need either biasing or heating. By using LF imaging, we demonstrate that this is due to a reduction of the molecular order whose impact is enhanced by the interpenetrating microphase-separated structures of the organic heterojunction, resulting in an increase of the electrical resistivity. The effect is well described as an increase in the Gaussian variance of the DOS in the framework of a Gaussian disorder model. High resolution, high write speed, low cost and low power consumption suggest this as a viable technique to be explored for several applications in polymer electronics. In particular, the technique could be optimized for the ultrahigh-density non-volatile data storage; in fact, by writing a feature of 20 nm as a basic bit, one would obtain a theoretical maximum data density of 1.6 Tb in −2 , exceeding the current technological limit, estimated in the range of 1 Tb in −2 . Of course, this practical application would need an optimization of the polymeric blend in several directions, trying to reduce all sources of noise when reading bits (hence, finding the best bias for reading, reducing the size of local conductivity inhomogeneity and so on) and looking for the blend preparation providing the optimal ‘writeability’, namely, best contrast between written and unwritten areas. Significant work should be done to assess long-term stability (months or more) and to develop a dedicated system exploiting our concept to store a significant amount of data. Nevertheless, the writing speed and the data density may represent a technological advantage with respect to other techniques being investigated, such as the electrostatic nanopatterning. Moreover, very modest forces are needed and no thermal excitation, making the principle viable for low power consumption systems. Importantly, the organic composite layer is inexpensive, easy to prepare, and to scale for very large areas. These features have to be kept in mind when considering challenges in terms of cost of recent promising techniques, as, for example, in the work by Cen et al . [24] , where the authors were able to exploit metal-insulator quantum phase transition at the interface between two insulating oxides to write conducting paths 3 nm wide. From a general point of view, our writing procedure may resemble to a standard mechanical indentation process, hence similar to the one proposed by Kim and collaborators [25] who reported that the baroplastic properties of block copolymers may be utilized to write bits (up to 1 Tb in −2 ) as depressed topographic features by an AFM tip. Incidentally, block copolymers are being actively investigated for mass memory device [26] , mostly owing to their self-assembly capabilities [27] . However, in our case the physical process is completely different, being induced by the sliding tip, and reading is not related to the detection of topographic depressions but only to changes in the conductivity. This observation also suggests further possible advantages, as reading of patterns is almost unrelated to topographic imperfections. As a matter of fact, an efficient AFM feedback is able to drive the tip on grains and surface imperfections and, as shown, for example, in Fig. 3 or Fig. 5 , the topography is generally not correlated with the conductivity map. In this way, requirements for surface flatness are mitigated. Moreover, the maximum achievable density of stored data would only be related to the size of the C-AFM tip, which in principle can be reduced to a few nanometres. Preparation of samples Two sets of P3HT alone and P3HT:[70]PCBM were prepared, namely, a first set (regioregularity: 95.7%; Mw: 65,200 g mol −1 ; polydispersity index: 2.2; mg content: 6 p.p.m. ; Ni content: <1 p.p.m.) and a second set (regioregularity: 95.2%; Mw: 36,600 g mol −1 ; polydispersity index: 2.0; mg content: 24 p.p.m. ; Ni content: 10 p.p.m.). Annealing was performed on a high-accuracy hot plate at 100°–140°–160°–200 °C for 15 s in ambient and rapidly quenched back to room temperature. ITO had a nominal surface resistivity of 15 Ohm per square . For both set of samples, a corresponding sample with an additional layer of poly(ethylene) dioxythiophene:poly(styrene) sulphonate (PEDOT:PSS) (47 nm) interposed between ITO and P3HT:[70]PCBM was prepared. No significant difference in the writing behaviour was observed in spite of a significant reduction in the surface roughness. Additional single-component and blend films were also prepared: F8BT:PCBM70 (1:1) as spun, on ITO, PDBTTT:PDI blend and PDBTTT alone. C-AFM measurements Measurements were performed either on air or saturated argon atmosphere by an NT-MDT Solver Pro P47 AFM, equipped with head for conductive, contact, semicontact and tapping measurements. In particular, the C-AFM measurements were realized by means of measuring head AU006. This is an adjustment unit for contact and resonant AFM, including the capability to measure current through conductive cantilever; the tip is kept at ground potential, whereas the sample is biased by a controlled voltage generator ( Fig. 1a ). Semicontact images were obtained by the same microscope. Several kinds of tips have been used: images shown in Fig. 3 have been obtained by the NSC19/Pt/no Al from Mikromasch. This is a silicon tip coated by 14 nm of Pt, featuring a curvature radius <24 nm and a typical force constant of 0.63 N m −1 (ranging between 0.17 and 1.7 N m −1 ). To evaluate the minimum interaction force, as detailed in the Supplementary Fig. S3 , we have used a softer tip, the CSC17/Pt/AlBS from Mikromasch, having a typical force constant 0.15 N m −1 (range 0.05–0.3 N m −1 ). Images in Figs 4 and 5 have been obtained by a tip NSC18/Pt, force constant 2.8 N m −1 (range 1.2–5.5 N m −1 ), radius <30 nm. Remaining scans were performed by NSC19-Ti/Pt, having the same features of the first set of tips, but exploiting an alloy of titanium/platinum as coating. Some additional tests (results not included) were performed by NSG03/Co/5 from NT-MDT, a tip featuring cobalt coating (typical k =1.1 N m −1 , range 0.5–2.2 N m −1 ), used to investigate and exclude the possible impact of the kind of conducting coating in the writing process. Extended Gaussian disorder model By numerically solving the master equation for hopping transport, assuming a disordered energy landscape with a Gaussian DOS, Pasveer et al. [16] have successfully determined the dependence of the charge carrier mobility for semiconductor polymers on temperature, carrier density and electric field. The results of the numerical solution of the master equation have been parameterized [16] , providing an approximation for the mobility: where in the above set of equations, c 1 =1.8 × 10 −9 and c 2 =0.42. Moreover, σ is the width of the Gaussian DOS (in eV), v 0 is the intrinsic hopping rate, a is an effective lattice constant, p the carrier density, e the electron charge, k B the Boltzmann’ constant and E the electric field. In this model, a and v 0 are fitting parameters along with the width of the Gaussian DOS. Generally, the carrier density p is function of the position x . To obtain the low-voltage IV curves, the above results are inserted in the expression here J is the current density, r is an estimated radius of the current-density spot, d is the thickness of the sample and ε is the dielectric constant. We still need the density of carriers p , which in turn is related to the electric field by the Gauss equation in [16] , the above equations are solved numerically. In our case, we have a thin film ( L =100–200 nm); to have a simple, closed form, approximation, we can assume the charge density to be spatially uniform so that the electric field is a linear function of space. In this way, the obtained value for the charge density can be seen as a space averaged effective value. In the limit of such an assumption, by integrating the electric field across the film to obtain the applied voltage, we can write p as the function of the applied voltage To compare the experimental data with the theory, measurements for P3HT:[70]PCBM were performed at relatively low voltages to avoid injection of electrons and measuring hole-only mobility. At low voltage, only positive carriers contribute to the current: in fact, based on the band structure shown in Fig. 1b , the ITO Fermi level lies just above the highest occupied molecular orbital energy level of P3HT and, hence, holes see a very low-energy barrier, easily overcome even with small biases. In particular, for positive (negative) voltages, holes are injected from the ITO electrode (Pt tip) to the Pt tip (ITO electrode) through the P3HT valence energy levels. At higher voltages, both positive and negative, also electrons can partially contribute to the current as they gain energy and can be injected over the forbidden gaps (of about 2 eV) of P3HT and PCBM. 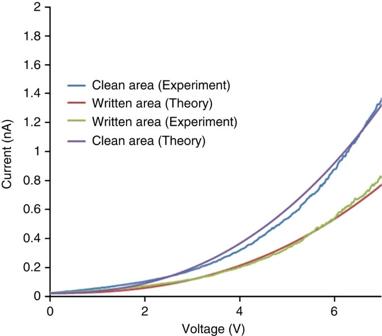Figure 6: EGDM model. Current–voltage characteristic as for P3HT:[70]PCBM annealed at 100 °C (blend involving higher Mw P3HT) for unwritten region and written region in same experiment, recorded at room temperature (T=300 K) and comparison with EGDM model. In the clean area, the width of the Gaussian DOS isσ=0.11 eV, whereasσ=0.116 eV in the written region. Experimental curves are average over five measurements. Figure 6 shows the comparison between the EGDM results (from the above equations) and data recorded at room temperature for the blend involving the higher Mw P3HT. EGDM fitting was obtained by selecting σ =0.11 eV for the clean area and σ =0.116 eV for the written area. Figure 6: EGDM model. Current–voltage characteristic as for P3HT:[70]PCBM annealed at 100 °C (blend involving higher Mw P3HT) for unwritten region and written region in same experiment, recorded at room temperature ( T =300 K) and comparison with EGDM model. In the clean area, the width of the Gaussian DOS is σ =0.11 eV, whereas σ =0.116 eV in the written region. Experimental curves are average over five measurements. Full size image How to cite this article: Farina, M. et al. Fast ultrahigh-density writing of low-conductivity patterns on semiconducting polymers. Nat. Commun. 4:2668 doi: 10.1038/ncomms3668 (2013).